Distinct axial and lateral interactions within homologous filaments dictate the signaling specificity and order of the AIM2-ASC inflammasome Inflammasomes are filamentous signaling platforms integral to innate immunity. Currently, little is known about how these structurally similar filaments recognize and distinguish one another. A cryo-EM structure of the AIM2 PYD filament reveals that the architecture of the upstream filament is essentially identical to that of the adaptor ASC PYD filament. In silico simulations using Rosetta and molecular dynamics followed by biochemical and cellular experiments consistently demonstrate that individual filaments assemble bidirectionally. By contrast, the recognition between AIM2 and ASC requires at least one to be oligomeric and occurs in a head-to-tail manner. Using in silico mutagenesis as a guide, we also identify specific axial and lateral interfaces that dictate the recognition and distinction between AIM2 and ASC filaments. Together, the results here provide a robust framework for delineating the signaling specificity and order of inflammasomes. Inflammasomes are filamentous signaling platforms and play key roles in the metazoan innate immune system [1] . These supra-structures assemble upon detecting molecular signatures arising from various intracellular catastrophes, such as genomic instability, dysfunctional organelles, and pathogen invasion [1] . Mammals have at least 15 different receptors that lead to the assembly of inflammasomes whose ultimate goal is to induce the polymerization of procaspase-1, activating the zymogen protease by proximity-induced autoproteolysis [1] . Caspase-1 then executes two key innate immune responses: the cleavage/maturation of pro-inflammatory cytokines, such as interleukin-1β and -18, and the initiation of pyroptosis [1] . Inflammasomes play essential roles in host defense against pathogen invasion (e.g., coronaviruses, herpesviridae, and Listeria monocytogene ) [1] , [2] , [3] , [4] , [5] , [6] . In addition, malfunctioning inflammasomes promote acute and chronic autoinflammatory diseases (e.g., severe COVID-19, rheumatoid arthritis, and systemic lupus erythematosus (SLE)) [7] , [8] , [9] , metabolic disorders (type 2 diabetes) [10] , [11] , and even tumorigenesis (colon cancer, lung cancer, and oral cancer) [12] , [13] . Inflammasome receptors contain multiple functional domains for autoinhibition, signal recognition, and oligomerization [1] , [14] . Importantly, the N-terminal pyrin domain (PYD) acts as the primary signal transduction module in the vast majority of inflammasomes [1] , [14] , [15] . PYDs are six-helix bundles that belong to the death-domain (DD) superfamily and can assemble into helical filaments. For instance, incoming signals such as viral nucleic acids induce the assembly of a receptor PYD filament [14] , [16] , [17] , [18] . The upstream PYD filaments then nucleate the filamentation of the PYD of central adaptor ASC (ASC PYD ) [14] , [18] , [19] , [20] , leading to the oligomerization of the CARD of ASC (ASC CARD ) to recruit and trigger the polymerization (activation) of procaspase-1 (ASC: apoptosis-associated speck-forming protein containing caspase-recruiting domain (CARD); CARDs are also six-helix bundles that belong to the DD family) [14] , [18] , [21] , [22] . Although the structural mechanisms by which inflammasomes assemble are increasingly better understood [14] , [17] , [18] , [19] , [20] , [21] , [22] , [23] , [24] , [25] , little is known about the mechanisms that direct the signaling order (sequence) and specificity. For instance, all published cryo-electron microscopy (cryo-EM) structures of PYD filaments show essentially the same helical architectures (six subunits per helical turn) [18] , [20] ; all CARD filaments also show the same helical architectures (four subunits per helical turn) [14] , [21] , [23] . These observations then led to a well-accepted model, in which the architectural complementarity between upstream and downstream filaments underpins the recognition [14] , [17] , [18] , [20] , [21] , [26] . However, it raises a considerably more complex problem as to how these similar helical filaments built from homologous protomers distinguish and recognize one another within respective subfamilies. Here, we address this fundamental mechanistic issue in the cytosolic double-stranded (ds)DNA-sensing AIM2-ASC inflammasome [27] . AIM2 (absent in melanoma 2) is a bipartite protein composed of the N-terminal PYD followed by the dsDNA-binding HIN domain (hematopoietic interferon-inducible nuclear antigen). Upon binding cytosolic dsDNA via its HIN domain, AIM2 PYD assembles into filaments, inducing the polymerization of ASC [12] , [16] , [17] , [19] . AIM2 is essential for the host defense against numerous pathogenic viruses and bacteria [6] , [12] , [16] , [27] , [28] , [29] , [30] . AIM2 also plays vital roles in neuronal development by regulating timely cell death [31] . However, dysregulated AIM2 leads to various maladies, such as SLE, chronic kidney diseases, and lung cancer [12] , [27] , [32] , [33] , [34] . We present a cryo-EM structure of the AIM2 PYD filament at 3.2 Å resolution, which reveals that its architecture is indeed identical to that of the ASC PYD filament. Using our structure, we then investigate how AIM2 PYD and ASC PYD filaments recognize, and distinguish each other by Rosetta and molecular dynamics (MD) simulations. Our in silico analyses consistently suggest that the energy landscapes that underpin the assembly of individual filaments do not impose directionality. By contrast, the energy landscape that governs the recognition between AIM2 PYD and ASC PYD is polarized in a head-to-tail manner. Multiple biochemical experiments corroborate that individual filaments assemble bidirectionally. Moreover, AIM2 PYD and ASC PYD filaments do not co-assemble, and the signal transduction from AIM2 to ASC occurs unidirectionally only when at least one is oligomeric. Using Rosetta-based in silico mutagenesis as a guide, our biochemical and cellular experiments consistently show that lateral interfaces of AIM2 PYD drive its bidirectional assembly. We also identify specific axial interfaces that mediate the recognition between AIM2 PYD and ASC PYD . Together, we demonstrate that distinct interfaces within homologous filaments direct signaling order and specificity of inflammasomes. We also set forth a broadly applicable multidisciplinary platform for delineating the signal transduction order, specificity, and directionality of filamentous assemblies. The cryo-EM structure of AIM2 PYD Using EM of negatively stained samples (nsEM), we previously found that the helical symmetry of the AIM2 PYD filament is consistent with that of the ASC PYD filament [17] , and thus proposed that architectural complementarity is important for their recognition. However, the published high-resolution cryo-EM structure of the AIM2 PYD filament displays an altered helical architecture because the N-terminal green fluorescence protein (GFP)-tag interferes with assembly [35] . Thus, we first determined the cryo-EM structure of the AIM2 PYD filament using an untagged recombinant protein. Cryo-EM images showed that AIM2 PYD filaments are straight helical rods (Fig. 1A ). The average power spectrum of 512-pixel-long nonoverlapping filament segments showed that the AIM2 PYD filament displays a six-start, C3 helical symmetry of 54.4° rotation (~6 subunits per helical turn) and an axial rise of 14 Å (Fig. 1B ). These parameters are remarkably similar to those of the ASC PYD filament [18] , further solidifying the concept that the upstream receptors provide structural templates for downstream assemblies in inflammasomes [14] , [17] , [26] . We fit the crystal structure of AIM2 PYD into the EM map for initial modeling [36] , and the refined high-resolution map allowed us to model in most bulky and aliphatic side chains (Fig. 1C ). The resolution of the final model was 3.2 Å according to the gold standard method (Supplementary Fig. 1A ). The diameter of the outer rim is ~94 Å and that of the inner cavity is ~25 Å (Fig. 1D ). The structure of individual AIM2 PYD protomers is identical to the crystal structure of AIM2 PYD monomer (Supplementary Fig. 1B ), thus indicating that, unlike the PYD of NLRP6 (ref. [20] ), an AIM2 PYD monomer does not undergo any conformational changes during activation. As seen from the ASC PYD filament, each AIM2 PYD subunit contributes three unique protein–protein interaction interfaces (Fig. 1E ). The type 1a:1b interface is largely composed of side-chain interactions, while the type 2a:2b and type 3a:3b interfaces involved both side-chain and backbone interactions (Fig. 1E ). We also noted several side chains previously implicated in filament assembly throughout different interfaces (e.g., L11, D19, F27, and I46; Fig. 1E ) [17] . Aligning the new AIM2 PYD filament to the GFP-AIM2 PYD filament demonstrates that although the lateral interactions are largely conserved, the axial positions are significantly different due to the altered helical symmetry (five subunits per turn in the GFP-tagged filament vs. six subunits per turn in the untagged filament; Supplementary Fig. 1C ). On the other hand, aligning the cryo-EM structures of AIM2 PYD and ASC PYD filaments demonstrates their congruent architectures (Fig. 1F ). The subtle difference in subunit positions between AIM2 PYD and ASC PYD filaments along the helical axis could reflect the unique side-chain interactions that mediate their respective filament assembly or the inherent flexibility of biomolecular structures (Fig. 1F ). Nevertheless, the near perfect architectural complementarity between AIM2 PYD and ASC PYD filaments supports the idea that upstream filaments provide structural templates for the assembly of downstream filaments [14] , [17] , [26] , [37] . Fig. 1: AIM2 PYD assembles into an architecturally congruent filament as the ASC PYD filament. A A sample cryo-electron micrograph of the AIM2 PYD filament (total 976 micrographs were taken). B An average power spectrum of the AIM2 PYD filament from 512 px-long nonoverlapping segments. C The AIM2 PYD filament model built into the EM map. A subunit with visible side chains is shown. D The model of AIM2 PYD filament. Each subunit is colored differently. E A cartoon representation of three unique filament interface types. Side chains at each filament interface are shown as a stick configuration. F Overlays between AIM2 PYD and ASC PYD (PDB ID: 3J63) filaments. Full size image Deciphering the specificity and directionality of the AIM2-ASC inflammasome using Rosetta and MD AIM2 PYD and ASC PYD monomers are homologous and structurally highly conserved (root-mean-squared-deviation, RMSD 0.5 Å), and our new cryo-EM structure shows that they indeed assemble into essentially identical filaments (Fig. 1F ). These observations raise significantly more complex questions as to whether and how these supra-structures distinguish and recognize each other. Importantly, such questions are germane to all filamentous signaling platforms employing PYDs or CARDs [21] , [22] , [26] , [37] , [38] , [39] . Thus, to establish a broadly relevant method for tackling these questions, we employed a computational approach using Rosetta. First, we tested whether RosettaDock [40] could recapitulate the cryo-EM structures by docking an AIM2 PYD monomer into our AIM2 PYD filament structure (also an ASC PYD monomer to the ASC PYD filament (PDB ID: 3J63) [18] ). For instance, each PYD protomer provides three unique interfaces in AIM2 PYD and ASC PYD filaments (i.e., six distinct surfaces; Figs. 1E and 2A ). To facilitate docking experiments, we generated a honeycomb-like side view of AIM2 PYD and ASC PYD filaments, in which the center protomer makes all six possible contacts (Fig. 2A ). We then divided the honeycomb into six unique subsections consisting of one ligand docked into a pocket created by three adjacent subunits (Fig. 2B ). Using the local docking method in Rosetta [40] , we performed 5000 independent docking simulations between a ligand–pocket pair from each subsection, then compared the interface energy and RMSD from the cryo-EM structures. Fig. 2: In silico studies suggest that homotypic filaments assemble bidirectionally and the recognition between AIM2 and ASC occurs unidirectionally. A Cartoon representations of honeycombs. Each interface type is labeled in the hexagons which represent PYD monomers. B Rosetta docking strategy. Top docking indicates that a ligand monomer docks onto the top surface of the pocket, while bottom docking is the opposite. C Plots of Rosetta interface energy scores vs. RMSD for top and bottom docking results for AIM2 PYD assembly. The B represents simulations conducted in C . D Plots of Rosetta interface energy scores vs. RMSD for docking an ASC PYD monomer on the top or bottom of AIM2 PYD pockets. E A model of the AIM2 PYD filament recognition of the ASC PYD filament. F , G Rosetta interface energy scores at individual filament interfaces for homotypic and heterotypic assemblies. AIM2 PYD -AIM2 PYD , ASC PYD -ASC PYD , ASC PYD -AIM2 PYD , and AIM2 PYD -ASC PYD . Each hexagon represents AIM2 PYD or ASC PYD monomer. H A plot for the difference in free energy (∆∆G) for dissociating ligand PYDs from the top or bottom pockets. Full size image For each filament, both parameters decreased concurrently, while displaying uniform energy scores from all subsections (Fig. 2C (arrow) and Supplementary Fig. 2A ), indicating that RosettaDock can recapitulate the cryo-EM structures. The more favorable energy scores from the AIM2 PYD filament suggest that it is is more stable than the ASC PYD filament (typically −70 s for AIM2 PYD complexes vs. −50 s for ASC PYD complexes). Importantly, the uniform energy scores throughout the top and bottom subsections (Fig. 2C and Supplementary Fig. 2A ) suggest that individual filaments would assemble bidirectionally. Next, we docked an ASC PYD monomer (ligand) onto all six pockets of the AIM2 PYD filament and vice versa (Fig. 2D and Supplementary Fig. 2B ). We first noted that the interface energies are not as favorable as the AIM2 PYD •AIM2 PYD complexes (−60 or worse for ASC PYD •AIM2 PYD complxes; Fig. 2D and Supplementary Fig. 2B ). Moreover, docking ASC PYD on the top pockets of the AIM2 PYD filament was significantly more favorable than docking at the bottom. (Fig. 2D orange vs. gray). Docking AIM2 PYD on the ASC PYD filament also showed that AIM2 PYD prefers the bottom half of the ASC PYD filament with the energy scores as favorable as the homotypic ASC PYD assembly (Supplementary Fig. 2A, B (2B orange vs. gray)). These results suggest that individual filaments assemble bidirectionally, while the recognition between AIM2 PYD and ASC PYD occurs unidirectionally, where the top of the AIM2 PYD filament recognizes the bottom of the ASC PYD filament (Fig. 2E ). Next, we used Rosetta InterfaceAnalyzer [41] to evaluate the interaction energies between homotypic and heterotypic interactions at the individual interfaces of the honeycomb (Fig. 2F ). The AIM2 PYD complex also showed the most favorable overall interface energy scores (Fig. 2G ). Moreover, for the respective homotypic assembly of AIM2 PYD and ASC PYD , the type 1 interface contributed most significantly with the top and bottom halves displaying symmetric energy scores (Fig. 2F ). On the other hand, the interface energy scores were consistently worse, when ASC PYD was placed at the center of the AIM2 PYD honeycomb, except for the one between the type 2a of ASC PYD and 2b of AIM2 PYD (Fig. 2F vs. 2G ). The overall energy scores between the top and bottom halves were again asymmetric, preferring a head-to-tail-like direction, in which the top of AIM2 PYD s favoring the bottom of ASC PYD and vice versa (Fig. 2E, G ; the small difference in energy scores between Fig. 2F, G likely stemmed from the subtle architectural differences in two filaments). To test whether the simulation results are not biased by a particular algorithm, we then used MD to calculate the free energy required to dissociate a ligand PYD from each pocket described in Fig. 2B (i.e., stability; Supplementary Fig. 2C, D ). Consistent with the results from RosettaDock, MD simulations suggested the AIM2 PYD filament complex to be most stable, followed by ASC PYD •AIM2 PYD then ASC PYD complexes. (Supplementary Fig. 3B ; see also Supplementary Fig. 3C for images showing the dissociation of each monomer before and after the simulation). We compared the sum of energies required to dissociate a ligand PYD from the top vs. bottom halves (Fig. 2H ; Supplementary Fig. 2C ). Individually, AIM2 PYD and ASC PYD complexes showed mostly uniform energy landscapes from either filament pole, with both filaments showing more stable interactions at the bottom (Fig. 2H and Supplementary Fig. 3A, B ). The moderate asymmetry suggests that the bottom interfaces might be preferred for homotypic assembly, or it could also reflect the intrinsic noise from sampling multiple conformations in an all-atom MD simulation. Nevertheless, consistent with Rosetta simulations, significantly more energy was required to dissociate ASC PYD from the top of the AIM2 PYD filament than the bottom (Fig. 2H and Supplementary Fig. 3B ). Together, our in silico analyses consistently suggest that individual filaments assemble bidirectionally, AIM2 PYD strongly prefers to assemble homotypically, and the recognition between AIM2 PYD and ASC PYD occurs via the type 2 interface. In vitro experiments corroborate in silico predictions To test our simulation results, we first tracked the assembly of fluor-labeled recombinant AIM2 PYD and ASC PYD filaments via confocal fluorescence microscopy. When we mixed two populations of differentially labeled maltose-binding-protein-tagged (MBP)-AIM2 PYD at 1:1 ratio and triggered polymerization by cleaving MBP via Tobacco Etch Virus protease (TEVp) [19] , the two colors colocalized in the same filaments (Fig. 3A , AIM2 PYD •AIM2 PYD ); differentially labeled ASC PYD populations also colocalized in the same filaments (Fig. 3A , ASC PYD •ASC PYD ). Importantly, when we preassembled the AIM2 PYD filament labeled with one color and added AIM2 PYD monomers labeled with a different color, nascent filaments extended from both axial poles of existing filaments (Fig. 3A , (AIM2 PYD filament) + AIM2 PYD ); ASC PYD filaments also displayed random bidirectional assembly (Fig. 3A , (ASC PYD filament) + ASC PYD ). These results corroborate that homotypic filaments assemble bidirectionally. Next, we mixed differentially labeled MBP-AIM2 PYD and MBP-ASC PYD at 1:1 ratio, and monitored their filament assembly upon triggering polymerization via TEVp. Here, each protein appeared to be oligomerized separately without colocalizing on the same filament, and two distinct filaments interacted only at one specific axial pole (Fig. 3B , AIM2 PYD •ASC PYD ). Such a unidirectional interaction was even more evident when we added excess nascent proteins over preformed filaments (Fig. 3B , (AIM2 PYD filament) + ASC PYD and (ASC PYD filament) + AIM2 PYD ). In addition, no significant Förster resonance energy transfer (FRET) signals were observed when we triggered the assembly of a donor-labeled AIM2 PYD and acceptor-labeled ASC PYD (Fig. 3C . see also ref. [19] ), indicating that AIM2 PYD and ASC PYD do not co-assemble, yet the recognition entails at least one to be oligomeric. Overall, our biochemical experiments agree with the computational predictions. Fig. 3: Individual filaments assemble bidirectionally and the recognition between AIM2 and ASC occurs at a specific pole. A Fluorescent confocal microscopy images of Alexa 488 - and Dylight 550 -labeled AIM2 PYD , Alexa 488 - and Dylight 550 -labeled ASC PYD , preassembled Alexa 488 -labeled AIM2 PYD filament and nascent Dylight 550 -labeled AIM2 PYD , and preassembled Alexa 488 -labeled ASC PYD filament and nascent Dylight 550 -labeled ASC PYD . B Fluorescent confocal microscopy images Alexa 488 -labeled AIM2 PYD and Dylight 550 -labeled ASC PYD , preassembled Alexa 488 -labeled AIM2 PYD filament and nascent Dylight 550 -labeled ASC PYD , and preassembled Alexa 488 -labeled ASC PYD filament and nascent Dylight 550 -labeled AIM2 PYD . Images shown in A and B are representatives of at least three independent experiments. C The time-dependent changes in FRET ratios between donor or acceptor-labeled MBP-AIM2 PYD and/or MBP-ASC PYD were monitored upon cleaving the MBP tag with TEVp. Full size image Simulations to identify key interfaces that govern the recognition and distinction between AIM2 PYD and ASC PYD Our observations thus far suggest that there exist distinct interactions that underpin individual assemblies and those that mediate the recognition between AIM2 PYD and ASC PYD , such as the type 2 interface for the heterotypic recognition. The side chains at the filament interfaces are poorly conserved between AIM2 PYD and ASC PYD (Supplementary Fig. 4A ), indicating that diverse side-chain interactions can support the assembly of homologous supra-structures (i.e., redundancy in assembly code). Thus, we decided to forego an alanine-scanning-like approach for identifying and validating key interfaces. Instead, we used Rosetta to suggest mutations that would selectively disrupt homotypic or heterotypic interactions without precluding filament assembly. Here, we in silico mutated each side chain of pocket protomers that interfaces ligand PYDs to all other a.a. using PyRosetta [42] (e.g., Fig. 4A top). We then obtained interface energy scores (∆Gs) for WT_ligand•WT_pocket and WT_ligand•mt_pocket complexes (Fig. 4A top. WT: wild type, mt: mutant); subtracting the ∆G of each WT•mt pair from that of the WT•WT pair then provided the effect of a given mutation (∆∆G). We then plotted ∆∆Gs for AIM2 PYD •AIM2 PYD (both top and bottom docking; Fig. 4A ) vs. ∆∆Gs for AIM2•ASC complexes (ASC PYD docking on the top pockets of AIM2 PYD ; Fig. 4A ). We found that the vast majority of mutations are deleterious for both AIM2 PYD •AIM2 PYD and AIM2 PYD •ASC PYD interactions (the upper right quadrant in Fig. 4A ), suggesting that the a.a. selection has already been optimized for the self-assembly and recognition. Nonetheless, we identified 88 mutations at nine unique side chains, resulting in ∆∆G (AIM2•AIM2) > 10 and ∆∆G (AIM2•ASC) < 10 (i.e., mutations that would selectively disrupt AIM2 PYD •AIM2 PYD interactions without abolishing AIM2 PYD •ASC PYD interactions; boxed area in Fig. 4B and listed in Supplementary Fig. 4B ). Interestingly, all these side chains were found on the lateral type 1 and type 3 interfaces, but none at the axial type 2 interfaces (Fig. 4B and Supplementary Fig. 4B ). Next, to identify mutations that would selectively disrupt AIM2 PYD •ASC PYD interactions, we looked for those resulted in ∆∆G (AIM2•AIM2) to be <10 and ∆∆G (AIM2•ASC) to be >10. Here, we identified 49 mutations at ten unique AIM2 PYD side-chain positions, all but one located on the type 2b surface (Fig. 4B and Supplementary Fig. 4B ). These results are consistent with the mechanism, in which the lateral interfaces drive the assembly of the AIM2 PYD filament without biasing any directions, while the recognition between AIM2 PYD and ASC PYD occurs at the type 2 interface. Fig. 4: in silico mutagenesis for identifying side chains that dictate the specificity of the AIM2-ASC inflammasome assembly. A Top: cartoons describing in silico mutagenesis strategy. The ligand monomer was kept WT and the interface residues of pocket monomers were mutated. The ∆∆G value for each mutated residue was obtained by ∆G (WT_ligand•WT_pocket) –∆G (WT_ligand•mt_pocket) . One pocket is shown as an example, and we applied the same strategy to all six pockets described in Fig. 2 (mt: mutant). Bottom: a plot of AIM2 PYD mutations that would interfere with AIM2 PYD •AIM2 PYD or AIM2 PYD •ASC PYD interaction. Selected mutations for follow-up biochemical and cellular studies are indicated. B A cartoon of the AIM2 PYD filament indicating the residues that Rosetta predicts to interfere with either homotypic assembly or ASC PYD recognition when mutated. Full size image In vitro and in cellulo experiments corroborate in silico predictions Mutations that abolish the self-assembly of AIM2 PYD decreases the dsDNA-binding activity of AIM2 FL , as oligomerization is couple to signal recognition [17] . Nevertheless, most of such AIM2 FL mutants still assemble into filaments on the dsDNA scaffold [17] . Also of note, AIM2 filaments can self-perpetuate its assembly by accelerating the polymerization of nascent monomers [19] . Thus, to test our simulation results, we generated Rosetta predicted mutations on AIM2 FL and first confirmed filament formation on dsDNA (Supplementary Fig. 5 ; all mutants formed filaments except N73L). We then determined whether dsDNA-bound AIM2 FL mutants could accelerate the polymerization of FRET donor/acceptor-labeled AIM2 PYD or ASC PYD (Fig. 5A–C and Supplementary Fig. 6 ; see also ref. [19] ) Fig. 5: biochemical and cellular experiments support Rosetta predictions. A Testing AIM2 FL mutants predicted to interfere with homotypic assembly. B Testing AIM2 FL mutants predicted to interfere ASC PYD recognition. C Testing ASC FL mutants predicted to interfere with AIM2 PYD recognition. For A – C , sample plots show the time-dependent polymerization of FRET donor- and acceptor-labeled AIM2 PYD or ASC PYD in the presence or absence of dsDNA-bound (linear plasmid ~5-kilo base-pairs (kbps)) WT or mutant AIM2 FL . Dot plots summarizing the effect of Rosetta predicted AIM2 mutants that would selectively interfere with its own assembly. Polymerization half-times were normalized using WT AIM2 FL -induced assembly (set to 1) and labeled PYDs alone (set to 0). * p < 0.05; ** p < 0.01; *** p < 0.001. P values were calculated using Student’s t test for paired samples. D Confocal microscope images of HEK293T cells (co)-transfected with WT ASC FL -mCherry alone. WT ASC FL -mCherry plus WT or mutant AIM2 FL -eGFP. E Confocal microscope images of HEK293T cells (co)-transfected with mutant ASC FL -mCherry plus WT AIM2 FL -eGFP. The nucleus is stained with DAPI in both D and E . Images shown in D and E are representative of at least three independent experiments. . Full size image As predicted from our simulation, L11A, A36D/R, and I46D were significantly more defective in accelerating the polymerization of AIM2 PYD than that of ASC PYD (Fig. 5A and Supplementary Fig. 6 ) We also tested D23K as it appeared to enhance the interaction with ASC, while disrupting AIM2–AIM2 interactions (Fig. 4A ). We found that D23K-AIM2 FL did not enhance the interaction with ASC PYD , but was more defective in inducing the polymerization of AIM2 PYD (Fig. 5A and Supplementary Fig. 6 ). These results consistently suggest that the lateral surface residues of AIM2 PYD preferentially, but not exclusively, promote homotypic assembly. Next, again consistent with Rosetta predictions, E21K and M75D were significantly more defective in inducing the polymerization of ASC PYD than that of AIM2 PYD (Fig. 5B and Supplementary Fig. 6 ), corroborating that the type 2b surface of the AIM2 PYD filament recruits ASC PYD (N73L-AIM2 FL failed to induce any filament formation consistent with the lack of self-assembly (Fig. 5 , and Supplementary Figs. 5 and 6 )). Notably, M75A-AIM2 FL (null in Rosetta mutagenesis) retained the WT-like activity (Supplementary Fig. 6 ), supporting the idea that a simple alanine-scanning approach is inadequate due to the redundancy in assembly code. We then used the above Rosetta-based approach to identify mutations at the type 2a surface of ASC PYD that would selectively disrupt the interaction with AIM2 PYD (Supplementary Fig. 7A–C ). Previously, we found that the ASC PYD filament accelerates the assembly of AIM2 PYD via a positive feedback loop [19] . Thus, we generated Rosetta predicted mutations on full-length ASC (ASC FL ) and tested their capacity for inducing the polymerization of FRET-labeled ASC PYD or AIM2 PYD . We used ASC FL , as the C-terminal CARD would promote the polymerization of ASC PYD even if mutations were too deleterious. We found that L61S and G37E were significantly more defective in accelerating the assembly of AIM2 PYD than that of ASC PYD , corroborating that the type 2a surface of ASC PYD recognizes AIM2 PYD (Fig. 5C and Supplementary Fig. 7D ). We next probe the interactions among AIM2 FL and ASC FL WT and mutants in HEK293T cells. WT AIM2 FL (ASC FL ) tagged with C-terminal eGFP or mCherry colocalized in the same complexes as expected (Supplementary Fig. 8 ). AIM2 FL showed filamentous complexes that often tangled up into speck-like clusters, while ASC FL displayed large puncta, as previously reported [43] (Fig. 5D left, Supplementary Fig. 8A–C ). AIM2 FL -eGFP mutants colocalized with WT AIM2 FL -mCherry (Supplementary Fig. 8B ), likely due to assembling/binding on the same (transfected) dsDNA strands as WT. Interestingly, when AIM2 FL -eGFP and ASC FL -mCherry were co-transfected, ASC FL filaments further expanded as if ASC FL assembles from multiple AIM2 FL foci (Fig. 5D , (+WT AIM2 FL )). When we co-transfected AIM2 FL -eGFP mutants and WT ASC FL -mCherry, those that preferentially decreased the ability to interact with AIM2 PYD still resulted in expanded ASC FL complexes as observed from WT (Fig. 5D , L11A, D23K, and A36D). By contrast, ASC FL stayed as a single punctum when co-transfected with AIM2 FL mutants that failed to accelerate the polymerization of ASC PYD (E21K and M75D; Fig. 5D , E21K and M75D); N73L-AIM2 FL -eGFP, which cannot oligomerize (Supplementary Figs. 5 and 8A ), also failed to interact with ASC FL -mCherry (Fig. 5D , N73L). We also imaged G37E- and L61S-ASC FL -mCherry with eGFP-tagged WT AIM2 FL and ASC FL . The ASC FL mutants still showed large puncta and also colocalized with WT (Supplementary Fig. 8C ). However, WT AIM2 FL -eGFP failed to colocalize or induce the expansion of these mutants when co-transfected (Fig. 5E ). Together, our in vitro and in cellulo experiments consistently support our in silico predictions, in which unique lateral and axial interfaces within homologous filaments dictate their recognition and distinction. Inflammasomes transduce signals by assembling supramolecular structures [14] , [17] , [18] , [19] , [20] , [22] , [23] . It is well accepted that architectural complementarity is important for the recognition between primary signaling components [21] , [22] , [23] , [28] , [30] , [34] . Indeed, our AIM2 PYD filament structure further cements this concept. Nevertheless, these observations further highlight a long-standing question as to how such homologous filaments distinguish and recognize one another. Here, we set forth a broadly applicable research platform for answering these questions and propose design principles that define the signaling mechanisms of inflammasomes. Strategies for homotypic filament assembly Our experiments consistently show that the assembly of individual filaments occur bidirectionally, with lateral type 1 and type 3 interfaces (especially type 1) of AIM2 PYD favoring homotypic interactions, while still supporting the recognition of ASC PYD . The lateral type 1 surfaces are the largest in any PYDs (Fig. 6A left), which would be ideal for recognizing other homotypic protomers to initiate assembly without any prescribed directionalities. The lack of directionality in homotypic assembly would then allow AIM2 to maximally benefit from one-dimensional random diffusion on pathogenic dsDNA [19] , resulting in a timely response by the upstream receptor (Fig. 6A right). Interestingly, the bidirectional assembly is in contrast to other cytoskeletal and signaling filaments such as actin [44] and B-cell lymphoma 10 (BCL10) [39] . Considering that both actin and BCL10 filaments originate from cell membranes/defined borders [39] , [44] , it is tempting to speculate that the bidirectional assembly of inflammasome filaments have evolved to take full advantage of no immediate boundaries in the cytosol. Fig. 6: Strategies for signal transduction by the AIM2-ASC inflammasome. A Left: a surface representation of AIM2 PYD monomer. The buried surface area in the filament for each interface type is indicated. Right: a scheme describing the advantages of bidirectional homotypic assembly. B The top surface view of the AIM2 PYD filament. Each solvent accessible interface is colored in red with the calculated surface area. C A scheme describing the advantages of unidirectional signal transduction by the AIM2-ASC inflammasome. Full size image Strategies for signaling by assembly The AIM2 PYD filament displays higher stability than either the ASC PYD filament or AIM2 PYD •ASC PYD complex (Fig. 2 ), which would ensure homotypic assembly of the receptor filament especially within the dsDNA scaffold. On the other hand, the interaction between AIM2 PYD and ASC PYD is more favorable than homotypic ASC PYD interactions at a specific axial pole (Fig. 2 ). In addition, AIM2 PYD and ASC PYD recognize each other only when at least one is oligomeric (Fig. 3B ). Of note, electrostatic surface analyses suggest that the charge complementary is reversed at the type 1 interface for AIM2 and ASC, likely indicating that the heterologous interactions between the monomers are not favorable (i.e., the type 1a surface of AIM2 PYD is largely basic, whereases that of ASC PYD is acidic; Supplementary Fig. 9A ). Importantly, our in silico, in vitro, and in cellulo experiments consistently demonstrate that the directional interaction at the type 2 interface is most critical (Figs. 2 – 5 ). The surface area of the type 2 interface is much smaller than that of the type 1 interface in monomeric PYDs (Fig. 6A ). However, because of the axial location, the type 2b surfaces become as accessible as the type 1 surfaces once AIM2 PYD assembles into a filament (Fig. 6B ). Moreover, electrostatic surface analyses suggest that the bottom of the AIM2 PYD filament is unfavorable for interacting with the ASC PYD filament due to highly positively charged surfaces (Supplementary Fig. 9B ). We propose that such conditional scaffolding by the upstream filament not only ensures proper signal transduction orders, but also maximizes signal amplification (Fig. 6C ). For instance, inflammasomes assemble in a digital fashion and entail cell death [14] , [19] . Thus, it must be imperative that ASC does not polymerize unless upstream receptors are fully activated by correct signals. Thus, the sequential/conditional assembly of the AIM2-ASC inflammasome would minimize its spurious activity in the absence of bona fide danger signals. Of note, not only the assembly, but also the signaling activity of AIM2 depends on dsDNA length, which regulates the probability of assembling the intact axial base of its filament [19] . Our results here further explain the dsDNA length-dependent mechanism, as the intact filament base would conditionally maximize the presence of the type 2b surfaces to recruit ASC (Fig. 6B ). Subsequently, such a stringent recognition mechanism would then ensure that ASC polymerizes homogenously via its prion-like assembly mechanism [45] , resulting in maximal signal amplification (Fig. 6C ). Alternatively, if AIM2 and ASC were to either co-assemble or interact without distinct energetic hierarchies, we envision that upstream and downstream oligomers would either alternate or even cap their respective assemblies, resulting in signal attenuation. Future directions Our successful implementation of Rosetta to decode the specificity of the AIM2-ASC inflammasome suggests that our approach can be broadly applied to other homologous signaling filaments. However, we noted that Rosetta was correct at ~50% in predicting energetically important mutations (Fig. 5 ), indicating that there is room for improvement. Nonetheless, given that precisely pinpointing the role of individual residues is intrinsically challenging, we find the Rosetta suite to be an excellent tool for decoding the specificity of the filamentous assemblies. It was recently postulated that the directionality of the NLRP6 PYD -ASC PYD interaction would be the same as what we found here for AIM2 PYD -ASC PYD (ref. [20] ). Thus, it is tempting to speculate that recruiting ASC via its type 2a surface by the type 2b surface of upstream receptors is the universal strategy in inflammasome signaling. Other than NLRP6 and AIM2, there are at least 14 other upstream receptors that signals through ASC [1] , [14] . Future investigations will reveal to what extent the mechanisms we found for AIM2 apply in other receptors and how well Rosetta fares in answering these questions. Protein expression and purification Human AIM2 FL (residues 1–343), AIM2 PYD (residues 1–94) S94C for fluorophore labeling, ASC PYD (residues 1–92) were cloned into the pET28b vector (Novagen) with an N-terminal MBP tag and TEVp recognition site. For cryo-EM, we and found a construct including ~20 a.a. in the unstructured linker region (residues 1–117) resulted in well-separated filaments (denoted as AIM2 IRND ; Fig. 1A ). ASC FL was cloned with the MBP tag at both N- and C-termini with the TEVp recognition site flanking MBP and ASC FL . All proteins were expressed in Escherichia coli BL21 Rosetta2 DE3 and purified using affinity (MBP/amylose), cation exchange, and followed by size-exclusion chromatography. Proteins were then concentrated and stored at −80 °C, see also refs. [17] , [19] (all primers generated for this study are listed in Supplementary Table 2 ). 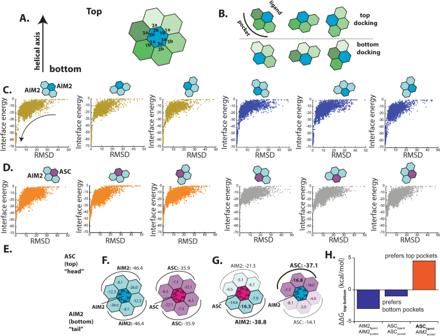Fig. 2: In silico studies suggest that homotypic filaments assemble bidirectionally and the recognition between AIM2 and ASC occurs unidirectionally. ACartoon representations of honeycombs. Each interface type is labeled in the hexagons which represent PYD monomers.BRosetta docking strategy. Top docking indicates that a ligand monomer docks onto the top surface of the pocket, while bottom docking is the opposite.CPlots of Rosetta interface energy scores vs. RMSD for top and bottom docking results for AIM2PYDassembly. TheBrepresents simulations conducted inC.DPlots of Rosetta interface energy scores vs. RMSD for docking an ASCPYDmonomer on the top or bottom of AIM2PYDpockets.EA model of the AIM2PYDfilament recognition of the ASCPYDfilament.F,GRosetta interface energy scores at individual filament interfaces for homotypic and heterotypic assemblies. AIM2PYD-AIM2PYD, ASCPYD-ASCPYD, ASCPYD-AIM2PYD, and AIM2PYD-ASCPYD. Each hexagon represents AIM2PYDor ASCPYDmonomer.HA plot for the difference in free energy (∆∆G) for dissociating ligand PYDs from the top or bottom pockets. Cryo-EM sample preparation A total of 5 µl sample of 2.75 µM AIM2 IRND (cleaved for 30 min with 6 µM TEVp) was applied to Lacey grids, followed by automatically blotting for 1.5 s and plunge freezing, using the FEI Vitrobot Mark IV operated at 100% humidity and room temperature (Johns Hopkins University). Cryo-EM data were collected at the National Cancer Institute National cryo-EM facility (NCI NCEF, Frederick, MD) using the FEI Titan equipped with the Gatan K2 direct electron detector operating at 300 keV, using the super-resolution mode (0.66 Å/pixel). A total of 2700 micrographs were collected from one grid at a defocus range from −1.0 to −2.5 µm. 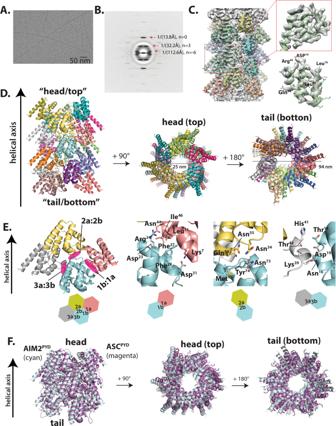Each micrograph was equally fractioned into 40 frames with a total exposure time of 12 s and a total dose of 42 electrons/Å 2 . Fig. 1: AIM2PYDassembles into an architecturally congruent filament as the ASCPYDfilament. AA sample cryo-electron micrograph of the AIM2PYDfilament (total 976 micrographs were taken).BAn average power spectrum of the AIM2PYDfilament from 512 px-long nonoverlapping segments.CThe AIM2PYDfilament model built into the EM map. A subunit with visible side chains is shown.DThe model of AIM2PYDfilament. Each subunit is colored differently.EA cartoon representation of three unique filament interface types. Side chains at each filament interface are shown as a stick configuration.FOverlays between AIM2PYDand ASCPYD(PDB ID: 3J63) filaments. Data collection statistics are listed in Supplementary Table 1 . Helical reconstruction and model building The 2700 micrographs were binned by two (to 1.32 Å/px) and frames were aligned using MotionCor2 (ref. [46] ). The defocus values and astigmatism of the micrographs were determined by CTFFIND3 for the aligned full-dose micrographs [47] . A total of 976 micrographs were selected (images with good CTF determination and defocus <3 μm) for subsequent image processing. CTF was corrected by multiplying the micrographs (only first 20 frames were aligned with a total dose of ~20 electrons/Å 2 ) with the theoretical CTF, which both corrects the phases and improves the signal-to-noise ratio. The e2helixboxer program in EMAN2 software package [48] was used for boxing long filaments from the full-dose images. The CTF-corrected micrographs were used for the segment extraction, with a total of 116,285 384 px-long overlapping segments (with a shift of 1.5 times of axial rise) generated. The SPIDER software package [49] was used for subsequent processing and reconstruction. Using a featureless cylinder as an initial reference, 99,237 segments were used in IHRSR program for the final reconstruction after the helical parameters (an azimuthal rotation of 53.3° and an axial rise of 14 Å per subunit) converged. The resolution of the final reconstruction was estimated by the FSC between two independent half maps, which shows 3.2 Å at FSC = 0.143. We used the crystal structure of AIM2 PYD (PDB ID: 4O7Q) as an initial template to dock into the AIM2 PYD cryo-EM map by rigid body fitting, and then manually edited the model in Chimera [50] and Coot [51] . We then used the modified model as the starting template to further refine against the segmented cryo-EM map using RosettaCM [52] . The refined monomeric model of AIM2 PYD was then rebuilt by RosettaCM with helical symmetry and real-space refined, using Phenix [53] to improve the stereochemistry, as well as the model-map correlation coefficient. The AIM2 PYD filament model was validated with MolProbity [54] . Refinement statistics are listed in Supplementary Table 1 . Rosetta docking The Rosetta Local Docking protocol [40] , [55] was applied to Rosetta symmetry relaxed structures of the AIM2 PYD cryo-EM structure and ASC PYD cryo-EM structure (PDB ID: 3J63). Each complex contained a pocket consisting of three PYDs, and one ligand PYD. The initial position of the ligand was already in the pocket to minimize the search space, as suggested by the local docking protocol. The docking simulation was done 5000 times for each fragment, and the results were analyzed by looking at the interface energy and RMSD from the initial position. Interface energy analysis and in silico mutagenesis We used the InterfaceAnalyzer script in Rosetta at individual interfaces of the honeycomb to obtain interaction energies. Using PyRosetta, we first in silico mutated each interface residue of all AIM2 PYD /ASC PYD protomers in the honeycomb into all other possible a.a. [42] . We then removed those that resulted in energy scores >2 standard deviations from the mean (e.g., prolines that would distort backbone geometry and cause potential folding issues). We then applied remaining mutants (942 possibilities) to the pocket protomers of all six subsections, leaving the ligand protomers as WT. We then used the dG_separate subroutine in Rosetta InterfaceAnalyzer to obtain ∆Gs for (WT_ligand•WT_pocket) and (WT_ligand•mutant_pocket) interfaces; subtracting the ∆G of each mutant from that of WT then provides the changes in interface energy caused by the mutation (∆∆G). Each mutant was tested at least three times and the average values were used for analyses. Molecular dynamics The coordinates for each protein–ligand complex were obtained from Rosetta docking experiments such that the interface energy score and interface RMSD were minimized. All MD simulations were performed using GROMACS 5.1.3 (gromacs.org) with an all-atom CHARMM36 (ref. [56] ) force field. Simulation scripts were created using CHARMM-GUI [57] , [58] . 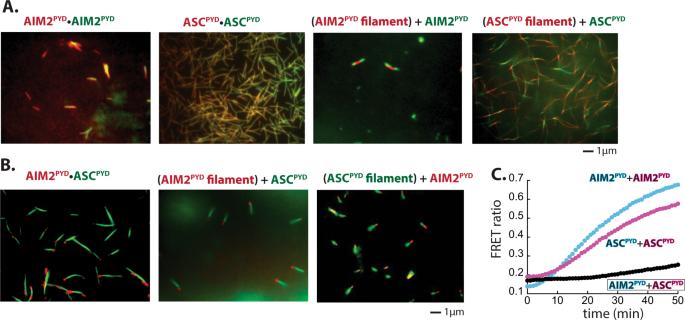Fig. 3: Individual filaments assemble bidirectionally and the recognition between AIM2 and ASC occurs at a specific pole. AFluorescent confocal microscopy images of Alexa488- and Dylight550-labeled AIM2PYD, Alexa488- and Dylight550-labeled ASCPYD, preassembled Alexa488-labeled AIM2PYDfilament and nascent Dylight550-labeled AIM2PYD, and preassembled Alexa488-labeled ASCPYDfilament and nascent Dylight550-labeled ASCPYD.BFluorescent confocal microscopy images Alexa488-labeled AIM2PYDand Dylight550-labeled ASCPYD, preassembled Alexa488-labeled AIM2PYDfilament and nascent Dylight550-labeled ASCPYD, and preassembled Alexa488-labeled ASCPYDfilament and nascent Dylight550-labeled AIM2PYD. Images shown inAandBare representatives of at least three independent experiments.CThe time-dependent changes in FRET ratios between donor or acceptor-labeled MBP-AIM2PYDand/or MBP-ASCPYDwere monitored upon cleaving the MBP tag with TEVp. Initial coordinates were energy minimized using the steepest descent algorithm and subsequently equilibrated for 4.75 ns, starting in the NVT ensemble and transitioning to the NPT ensemble. Neutralizing ions were added with ~200 Cl and ~200 K to a box of 13 nm × 13 nm × 13 nm. Following initial energy minimization and equilibration, a second step of equilibration was performed in the NPT ensemble with a 2 fs timestep for 50 ns. A Nose-Hoover [59] thermostat was used to maintain a reference temperature of 300 K with a 1 ps coupling time constant. The protein and solvent were coupled to separate temperature baths. A Parrinello-Rahman [6] isotropic barostat with a 5 ps coupling time constant was used to maintain a pressure of 1 bar. Particle Mesh Ewald (PME) with a 1.2 nm cutoff radius, a 0.12 nm Fourier spacing, and cubic interpolation of 4 were used for electrostatics [60] . Van der Waals interactions had a 1.2 nm cutoff radius. A LINCS algorithm was used for bond constraints and XYZ periodic boundary conditions were enforced [61] . Following the second step of equilibration, well-tempered Metadynamics (MetaD) simulations were performed using GROMACS 5.1.3 patched with PLUMED2 (ref. [62] ), using a CHARMM36 force field. The collective variable (CV) was the distance between the center-of-mass of the pocket and the center-of-mass of the ligand (residue 60). The backbone RMSD stayed mostly constant during the course of simulation (Supplementary Fig. 3A ). Gaussians of energy were deposited along the trajectory in this CV space. Gaussians had an initial hill height of 1 kJ/mol and a width of 0.05 nm. Gaussians were deposited every 400 fs. A bias factor of 4 was used to adjust the hill heights according to the well-tempered MetaD scheme. Gaussians were saved to a grid with a bin spacing 0.01 nm. Simulations were considered complete when the ligand completely dissociated from the pocket, i.e., the CV distance exceeded 5 nm. Positional restraints were placed on every alpha-carbon in the pocket to prevent dissociation of the pocket protomers during the entirety of the MetaD simulations. The sum of all deposited Gaussians was computed to represent the dissociation free energy. Polymerization assays A total of 100 nM of AIM2 FL was cleaved by 6 µM TEVp for 20 min in a 384-well plate. After cleavage, 150 nM of linearized plasmid dsDNA (~5-kbps, binding site normalized) was added and allowed to bind for 30 min. To start the assay, 2 µM FRET mix of MBP-tagged AIM2 PYD or ASC PYD was added to the same well containing TEVp. Each experiment consisted of a control well with no AIM2 FL , one with AIM2 FL WT, and multiple AIM2 FL mutants for both AIM2 PYD and ASC PYD wells. AIM2 and ASC samples were run at the same time to ensure proper statistical analyses. Half-times for polymerization were calculated and converted to apparent kinetic rates [19] , [63] . The no AIM2 FL control and AIM2 FL WT control were used to normalize the kinetics rates for each mutant into an activity ratio scaling from 0 (no AIM2 FL present) to 1 (AIM2 FL WT activity). P values were calculated using Student’s t test for paired samples. The same strategy was used for ASC FL WT and mutants (0.5 µM, precleaved by TEVp for 30 min) inducing the polymerization of FRET-labeled AIM2 PYD or ASC PYD . nsEM AIM2 FL bound to dsDNA was prepared in the same manner as for the polymerization assays (100 nM protein, 150 nM dsDNA, linear plasmid ~5 kilo-bps). The samples were applied to carbon coated grids and imaged [19] , [64] . Imaging recombinant AIM2 PYD and ASC PYD filaments Filament assembly of Alexa 488 - or Dylight 550 -labeled MBP-AIM2 PYD and MBP-ASC PYD (1 µM each or 3 µM of nascent proteins for Fig. 3A ) was induced by removing MBP by TEVp as indicated in figure legends. For preassembly, the AIM2 PYD or ASC PYD filament was cleaved and incubated for 30 min prior to adding nascent proteins. 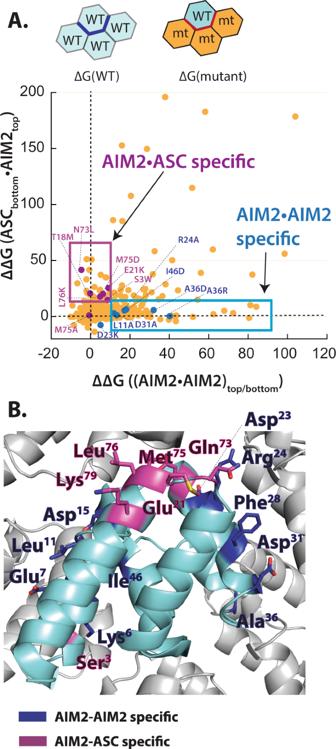Fig. 4: in silico mutagenesis for identifying side chains that dictate the specificity of the AIM2-ASC inflammasome assembly. ATop: cartoons describing in silico mutagenesis strategy. The ligand monomer was kept WT and the interface residues of pocket monomers were mutated. The ∆∆G value for each mutated residue was obtained by ∆G(WT_ligand•WT_pocket)–∆G(WT_ligand•mt_pocket). One pocket is shown as an example, and we applied the same strategy to all six pockets described in Fig.2(mt: mutant). Bottom: a plot of AIM2PYDmutations that would interfere with AIM2PYD•AIM2PYDor AIM2PYD•ASCPYDinteraction. Selected mutations for follow-up biochemical and cellular studies are indicated.BA cartoon of the AIM2PYDfilament indicating the residues that Rosetta predicts to interfere with either homotypic assembly or ASCPYDrecognition when mutated. Images were then taken using a Zeiss Axioskop 50 with a Zeiss Axiocam HRC camera and an Axio Observer inverted microscope with LSM700 confocal module. Imaging AIM2 FL -eGFP/mCherry and ASC FL -eGFP/mCherry in HEK293T cells AIM2 FL and ASC FL variants were cloned into the pCMV6 vector harboring eGFP or mCherry. To preserve native PYD–PYD interactions, the fluorescent proteins were positioned at the C-terminus of AIM2 FL or ASC FL . Plasmids were then transiently transfected into HEK293T cells using lipofectamine (0.5 µg each plasmid; Invitrogen). 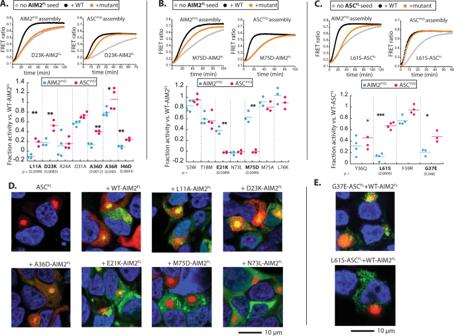Fig. 5: biochemical and cellular experiments support Rosetta predictions. ATesting AIM2FLmutants predicted to interfere with homotypic assembly.BTesting AIM2FLmutants predicted to interfere ASCPYDrecognition.CTesting ASCFLmutants predicted to interfere with AIM2PYDrecognition. ForA–C, sample plots show the time-dependent polymerization of FRET donor- and acceptor-labeled AIM2PYDor ASCPYDin the presence or absence of dsDNA-bound (linear plasmid ~5-kilo base-pairs (kbps)) WT or mutant AIM2FL. Dot plots summarizing the effect of Rosetta predicted AIM2 mutants that would selectively interfere with its own assembly. Polymerization half-times were normalized using WT AIM2FL-induced assembly (set to 1) and labeled PYDs alone (set to 0). *p< 0.05; **p< 0.01; ***p< 0.001.Pvalues were calculated using Student’sttest for paired samples.DConfocal microscope images of HEK293T cells (co)-transfected with WT ASCFL-mCherry alone. WT ASCFL-mCherry plus WT or mutant AIM2FL-eGFP.EConfocal microscope images of HEK293T cells (co)-transfected with mutant ASCFL-mCherry plus WT AIM2FL-eGFP. The nucleus is stained with DAPI in bothDandE. Images shown inDandEare representative of at least three independent experiments. . 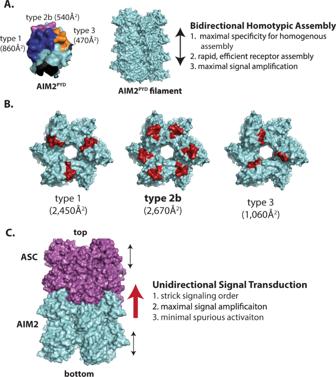Fig. 6: Strategies for signal transduction by the AIM2-ASC inflammasome. ALeft: a surface representation of AIM2PYDmonomer. The buried surface area in the filament for each interface type is indicated. Right: a scheme describing the advantages of bidirectional homotypic assembly.BThe top surface view of the AIM2PYDfilament. Each solvent accessible interface is colored in red with the calculated surface area.CA scheme describing the advantages of unidirectional signal transduction by the AIM2-ASC inflammasome. After 12 h, cells were fixed with 4% paraformaldehyde and mounted on glass slides using ProLong Gold Antifade Mountant with DAPI (Thermo Fisher). Cells were then imaged using the same confocal microscope as the recombinant proteins. Reporting summary Further information on research design is available in the Nature Research Reporting Summary linked to this article.